A distinct sodium channel voltage-sensor locus determines insect selectivity of the spider toxin Dc1a β-Diguetoxin-Dc1a (Dc1a) is a toxin from the desert bush spider Diguetia canities that incapacitates insects at concentrations that are non-toxic to mammals. Dc1a promotes opening of German cockroach voltage-gated sodium (Na v ) channels (BgNa v 1), whereas human Na v channels are insensitive. Here, by transplanting commonly targeted S3b–S4 paddle motifs within BgNa v 1 voltage sensors into K v 2.1, we find that Dc1a interacts with the domain II voltage sensor. In contrast, Dc1a has little effect on sodium currents mediated by PaNa v 1 channels from the American cockroach even though their domain II paddle motifs are identical. When exploring regions responsible for PaNa v 1 resistance to Dc1a, we identified two residues within the BgNa v 1 domain II S1–S2 loop that when mutated to their PaNa v 1 counterparts drastically reduce toxin susceptibility. Overall, our results reveal a distinct region within insect Na v channels that helps determine Dc1a sensitivity, a concept that will be valuable for the design of insect-selective insecticides. Insect voltage-gated sodium (Na v ) channels share a common architecture with their mammalian orthologues [1] . The pore-forming subunit consists of four connected domains (DI–IV), each with six transmembrane segments (S1–S6). These homologous, but not identical, domains each contain a voltage sensor (S1–S4) and a portion of the pore through which Na + can diffuse (S5–S6) [2] . While they have yet to be identified in insect Na v channels, each voltage-sensing domain within mammalian and bacterial Na v channels contains an S3b–S4 helix-turn-helix motif, the voltage-sensor paddle, which drives voltage-sensor activation [3] , [4] , [5] , [6] . Aside from its vital role in channel gating, the paddle motif is also an important pharmacological target, as peptide toxins interact with this region to modify channel opening [3] , [4] , [7] . Insect Na v channels likely possess similar motifs since residue substitutions in homologous regions can abolish channel susceptibility to toxins found in animal venoms [1] . Even though voltage-sensing domains are extensively targeted by naturally occurring peptides, commercially available insecticides such as pyrethroids and oxadiazines typically interact with the channel pore region or intracellular linker between S4 and S5 to disrupt opening or closing (that is, gating) [8] , [9] . However, insects have responded to this threat by mutating residues at strategic locations within the channel that result in a reduced sensitivity to these compounds [9] . Moreover, the conserved nature of the Na v channel pore throughout the animal kingdom often leads to undesired biological activity of insecticides in beneficial insect orders or mammals [8] , [9] , [10] . Since the amino acid composition of voltage-sensing domains varies considerably between related Na v channel isoforms, these regions may replace the pore as a target for designing insecticides with a higher degree of phyletic selectivity, an intriguing notion that has yet to be fully explored. Na v channels have been governing electrical excitability in a wide range of organisms for millions of years, even before the development of neurons [2] , [11] . Thus, it is not surprising that ancient organisms such as spiders developed an arsenal of toxins geared towards incapacitating prey by modulating Na v channel function [12] , [13] , [14] , [15] . One intriguing specimen is the desert bush spider ( Diguetia canities ) whose habitat spans the Southwestern deserts of the United States [16] , [17] . The venom of this relatively unexplored primitive weaving spider contains a 57-residue peptide known as DTX9.2 (or β-diguetoxin-Dc1a [18] , hereafter Dc1a; Fig. 1a ), one of the most potent insect-selective neurotoxins found in arthropod venoms [19] . Although its precise molecular target has yet to be elucidated, neurophysiological studies on housefly larvae revealed excitation of sensory and neuromuscular preparations on Dc1a application that could be blocked by the Na v channel-blocking compound tetrodotoxin [20] . 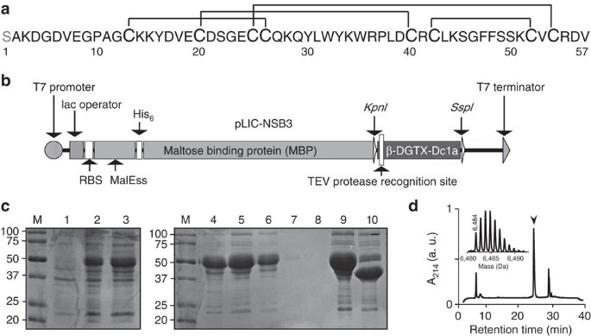Figure 1: Recombinant production of Dc1a. (a) Primary structure of rDc1a. The non-native N-terminal Ser residue that is a vestige of the TEV protease cleavage site used for recombinant toxin production is highlighted in grey. Disulphide bridge connectivity is shown above the sequence. (b) Schematic representation of the pLIC-NSB3 vector used for periplasmic expression of rDc1a. The coding region includes a MalE signal sequence (MalESS) for periplasmic export, a His6affinity tag, an MBP fusion tag and a codon-optimized gene encoding rDc1a, with a TEV protease recognition site inserted between the MBP and toxin-coding regions. The locations of key elements of the vector are shown, including the ribosome-binding site (RBS). (c) SDS-polyacrylamide gel electrophoresis gels illustrating different steps in the purification of rDc1a. Lanes contain: M, molecular weight markers; lane 1,E. colicell extract before IPTG induction; lane 2,E. colicell extract after IPTG induction; lane 3, soluble periplasmic extract (the His6-MBP-rDc1a fusion protein is evident at ~50 kDa); lane 4, Ni-NTA beads after loading the cell lysate; lane 5, eluate-1 from washing Ni-NTA resin with 600 mM imidazole; lane 6, elute-2 from washing Ni-NTA resin with 600 mM imidazole; lane 7, eluate-3 from washing Ni-NTA resin with 600 mM imidazole; lane 8, Ni-NTA beads after elution-3; lane 9, fusion protein sample before TEV protease cleavage; lane 10, fusion protein sample after TEV protease cleavage showing almost complete cleavage of fusion protein to His6-MBP. (d) RP-HPLC chromatogram showing the final step in the purification of rDc1a. The arrow head denotes the peak corresponding to correctly folded recombinant rDc1a. Inset is a MALDI-TOF MS spectrum showing the [M+H]+ion for the purified recombinant toxin (obs.=6,484 Da; calc.=6,485.39 Da). Figure 1: Recombinant production of Dc1a. ( a ) Primary structure of rDc1a. The non-native N-terminal Ser residue that is a vestige of the TEV protease cleavage site used for recombinant toxin production is highlighted in grey. Disulphide bridge connectivity is shown above the sequence. ( b ) Schematic representation of the pLIC-NSB3 vector used for periplasmic expression of rDc1a. The coding region includes a MalE signal sequence (MalE SS ) for periplasmic export, a His 6 affinity tag, an MBP fusion tag and a codon-optimized gene encoding rDc1a, with a TEV protease recognition site inserted between the MBP and toxin-coding regions. The locations of key elements of the vector are shown, including the ribosome-binding site (RBS). ( c ) SDS-polyacrylamide gel electrophoresis gels illustrating different steps in the purification of rDc1a. Lanes contain: M, molecular weight markers; lane 1, E. coli cell extract before IPTG induction; lane 2, E. coli cell extract after IPTG induction; lane 3, soluble periplasmic extract (the His 6 -MBP-rDc1a fusion protein is evident at ~50 kDa); lane 4, Ni-NTA beads after loading the cell lysate; lane 5, eluate-1 from washing Ni-NTA resin with 600 mM imidazole; lane 6, elute-2 from washing Ni-NTA resin with 600 mM imidazole; lane 7, eluate-3 from washing Ni-NTA resin with 600 mM imidazole; lane 8, Ni-NTA beads after elution-3; lane 9, fusion protein sample before TEV protease cleavage; lane 10, fusion protein sample after TEV protease cleavage showing almost complete cleavage of fusion protein to His 6 -MBP. ( d ) RP-HPLC chromatogram showing the final step in the purification of rDc1a. The arrow head denotes the peak corresponding to correctly folded recombinant rDc1a. Inset is a MALDI-TOF MS spectrum showing the [M+H] + ion for the purified recombinant toxin (obs.=6,484 Da; calc.=6,485.39 Da). Full size image Here, we show that Dc1a potently promotes opening of the German cockroach Na v channel BgNa v 1 (ref. 21 ) by interacting with the paddle motif in domain II. Surprisingly, Dc1a has little effect on PaNa v 1-expressing neurons isolated from the American cockroach ( Periplaneta americana ) [22] , even though the toxin-binding site is identical in these two cockroach channels. By exploring regions responsible for the remarkable insect-family specificity of Dc1a, we uncovered an important role for the domain II S1–S2 loop in determining PaNa v 1 resistance to Dc1a. Together with the unique solution structure of Dc1a, our results provide a proof of concept that toxins—and by extension small molecules—can selectively target insect Na v channels by interacting with their voltage-sensing domains, thus facilitating the development of new insecticides. Production of recombinant Dc1a We first produced recombinant Dc1a peptide (rDc1a) using a novel approach that addresses the challenge of correctly folding disulphide-rich spider toxins in E. coli [23] . To this end, we created an isopropyl-β-D-thiogalactopyranoside (IPTG)-inducible construct ( Fig. 1b ) that allows for export of a His 6 -MBP-Dc1a fusion protein to the E. coli periplasm, where the enzymes involved in disulphide-bond formation are located [23] . On recovery from the soluble cell fraction, the fusion protein was purified using nickel affinity chromatography ( Fig. 1c ). Subsequent cleavage and chromatographic purification yielded a single major disulphide-bond isomer with a purity of >98% as assessed by SDS-polyacrylamide gel electrophoresis and matrix-assisted laser desorption/ionization time-of-flight (MALDI-TOF) mass spectrometry ( Fig. 1d ). Note that, with four disulphide bonds, there are 105 possible disulphide-bond isomers of rDc1a. Overall, the final yield was ~1.1 mg of toxin per litre of culture. Since native Dc1a was unavailable to us, we confirmed the insecticidal activity of rDc1a by injection into the blowfly Lucilia cuprina and the housefly Musca domestica , which yielded LD 50 values of 231±32 pmol g −1 and 493±52 pmol g −1 , respectively ( n =3) ( Supplementary Fig. 1 ). We therefore conclude that rDc1a has a similar lethality to agricultural pests when compared with native toxin [19] . Solution structure of rDc1a The development of an efficient bacterial expression system allowed us to produce uniformly 13 C/ 15 N-labelled rDc1a protein for structure determination using heteronuclear NMR. 1 H N , 15 N, 13 C α , 13 C β , and 13 C′ resonance assignments for the toxin were obtained from analysis of amide-proton strips in three-dimensional (3D) HNCACB, CBCA(CO)NH, and HNCO spectra. Sidechain 1 H and 13 C chemical shifts were obtained using a four-dimensional (4D) HCC(CO)NH-TOCSY experiment, which has the advantage of providing sidechain 1 H– 13 C connectivities [24] . Complete chemical shift assignments have been deposited in BioMagResBank (Accession Number 19666 ). CYANA was used for automated NOESY assignment and structure calculation [25] . The disulphide-bond pattern (1–4, 2–5, 3–8, 6–7) was unambiguously determined from preliminary structures calculated without disulphide-bond restraints [26] and is identical to the framework predicted in the UniProtKB entry for Dc1a (P49126). Of the 200 structures that were calculated from random starting conformations, 20 conformers with high stereochemical quality (as judged by MolProbity [27] ) were selected to represent the solution structure of rDc1a ( Fig. 2a ). Atomic coordinates for the final ensemble of 20 structures are available from the Protein Data Bank (PDB; Accession Number 2MI5 ). 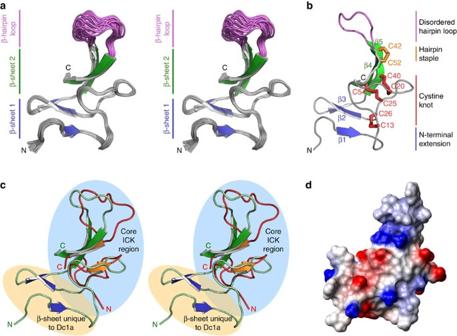Figure 2: NMR solution structure of rDc1a. (a) Stereo view of the ensemble of 20 rDc1a structures. The structures are overlaid over the backbone atoms of residues 2–42 and 52–56 in order to highlight the disordered nature of the hairpin loop (residues 43–51, purple) relative to the well-structured ICK region of the toxin. The N and C termini are labelled and the β-strands that form the N- and C-terminal β-sheets are coloured blue and green, respectively. (b) Ribbon representation of rDc1a highlighting the five β- strands (β1–β5) and four disulphide bonds. The three disulphide bonds that form the ICK motif are shown in red while the fourth disulphide that staples the base of the disordered β4–β5 hairpin loop is highlighted in orange. The β-strands and disordered hairpin loop are coloured as ina. (c) Stereo view of the structures of As1a, a typical knottin peptide30, overlaid with rDc1a. The two structures were overlaid for optimal superposition over their core ICK regions (28 residues; region highlighted in cyan) using the CLICK server70. Note that the N-terminal β-sheet in rDc1a is quite distinct from the region of structural overlap. (d) Electrostatic surface potential of rDc1a with positive and negative charges shown in blue and red, respectively. The molecular orientation is the same as in panelsaandc. Figure 2: NMR solution structure of rDc1a. ( a ) Stereo view of the ensemble of 20 rDc1a structures. The structures are overlaid over the backbone atoms of residues 2–42 and 52–56 in order to highlight the disordered nature of the hairpin loop (residues 43–51, purple) relative to the well-structured ICK region of the toxin. The N and C termini are labelled and the β-strands that form the N- and C-terminal β-sheets are coloured blue and green, respectively. ( b ) Ribbon representation of rDc1a highlighting the five β- strands (β1–β5) and four disulphide bonds. The three disulphide bonds that form the ICK motif are shown in red while the fourth disulphide that staples the base of the disordered β4–β5 hairpin loop is highlighted in orange. The β-strands and disordered hairpin loop are coloured as in a . ( c ) Stereo view of the structures of As1a, a typical knottin peptide [30] , overlaid with rDc1a. The two structures were overlaid for optimal superposition over their core ICK regions (28 residues; region highlighted in cyan) using the CLICK server [70] . Note that the N-terminal β-sheet in rDc1a is quite distinct from the region of structural overlap. ( d ) Electrostatic surface potential of rDc1a with positive and negative charges shown in blue and red, respectively. The molecular orientation is the same as in panels a and c . Full size image Statistics highlighting the high precision and stereochemical quality of the ensemble of rDc1a structures are shown in Supplementary Table 1 . The average MolProbity score of 1.24 places the ensemble in the 99th percentile relative to all other structures ranked by MolProbity. The high stereochemical quality of the ensemble stems from a complete absence of bad close contacts and an excellent Ramachandran plot quality (>99% of residues in the most favoured region). The structural ensemble is also highly precise with backbone and heavy-atom root-mean-square deviation (r.m.s.d.) values over all the structural ordered regions (residues 3–42, 52–56) of 0.27±0.07 Å and 0.70±0.11 Å, respectively. The ensemble of rDc1a structures ranks as ‘very high resolution’ based on these measures of precision and stereochemical quality [28] . Three of the four disulphide bonds in rDc1a form a classical inhibitor cysteine knot (ICK) motif in which the Cys13–Cys26 and Cys20–Cys40 disulphide bonds and the intervening sections of the polypeptide backbone form a 23-residue ring that is pierced by the Cys25–Cys54 disulphide bond ( Fig. 2b ). This ICK motif is commonly found in spider toxins, and this particular scaffold provides these peptides (so-called `knottins') with an unusually high degree of chemical, thermal and biological stability [15] . However, the structure of rDc1a differs markedly from other ICK toxins, and a DALI search [29] of the PDB returned no structural homologues. First, rDc1a contains an additional disulphide bond (Cys42–Cys52) that appears to serve as a molecular staple which limits the flexibility of a disordered serine-rich hairpin loop (residues 43–51) ( Fig. 2b ). Stapled hairpins of this kind have been observed in only a small number of spider toxins [30] . Second, the extended N terminus of rDc1a along with an unusually large loop between Cys26 and Cys40 enables the formation of an amino-terminal (N-terminal) three-stranded antiparallel β-sheet that is not found in any other knottin ( Fig. 2b,c ). The uniqueness of the rDc1a structure can readily be seen by comparison with the structure of As1a, a typical spider venom–derived knottin that modulates the activity of insect Na V channels [30] . The two toxins can be aligned over their core ICK regions with an rmsd of 1.9 Å ( Fig. 2c ) consistent with them both being members of the knottin family. However, when aligned over this ICK region, the N-terminal β-sheet of rDc1a is entirely separate to the region of structural overlap ( Fig. 2c ). Despite its structural uniqueness, the molecular surface of rDc1a contains a relatively uniform distribution of charged residues ( Fig. 2d ); moreover, there are no distinct clusters of hydrophobic residues that might mediate an interaction with lipid bilayers [7] , [31] ( Supplementary Movie 1 ). rDc1a opens the German cockroach Na v channel BgNa v 1 Diguetia spiders are generalist predators and their diet consists of various insects ranging from small ants to sizeable prey such as grasshoppers and cockroaches [16] , [32] . As such, we decided to test whether rDc1a influences the gating properties of BgNa v 1, a well-studied Na v channel isoform cloned from the German cockroach [8] , [21] . We functionally expressed BgNa v 1 in Xenopus oocytes and applied various concentrations of rDc1a. At 1 μM, rDc1a produced robust opening of BgNa v 1 at voltages where the channel is normally closed. This was achieved by a drastic shift in channel activation to more negative potentials (V 1/2 was shifted from −27.3±0.2 mV (mean±s.e.m.) (slope 4.0±0.2) to −49.4±0.4 mV (slope 3.5±0.3) in the presence of 1 μM rDc1a; Fig. 3a ) whereas steady-state inactivation (or channel availability) was only slightly affected (V 1/2 was shifted from −52.2±0.1 mV to −55.1±0.1 mV in the presence of 1 μM rDc1a; Fig. 3a ). The rate of recovery from fast inactivation was also not significantly altered ( τ is 2.1±0.1 ms versus 2.2±0.1 ms; Fig. 3b ). On addition of 1 μM rDc1a to channels depolarized to −60 mV every 5 s, sodium currents became rapidly visible as a result of the −22 mV shift in voltage-dependent opening of BgNa v 1 ( Fig. 3c ). Moreover, rDc1a similarly affects the channel when voltage-steps to −60 mV were applied every 50 s, suggesting that the toxin can access its binding site when BgNa v 1 is in the resting state [12] . Channels completely recovered following washout in toxin-free solution ( Fig. 3c ). The persistent nature of the emerging current does not stem from the inhibition of fast inactivation by rDc1a since wild-type (WT) BgNa v 1 inherently possesses these characteristics at mildly depolarizing voltages [33] . Fitting the Hill equation to the concentration dependence for toxin-induced current potentiation, as determined by shifts in V 1/2 , yielded an EC 50 of 65±1 nM and a Hill coefficient of 1.19±0.02 ( Fig. 3d ), suggesting that the toxin may interact with only one binding site. 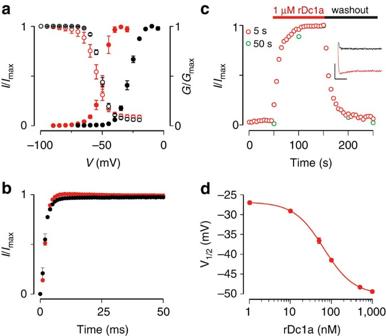Figure 3: rDc1a promotes opening of BgNav1 channels. (a) Comparison of the gating properties of BgNav1 before (black), and after (red), addition of 1 μM rDc1a. Shown are the normalized deduced conductance (G)–voltage (filled circles) (G/Gmax) and steady-state inactivation (open circles;I/Imax) relationships. Currents were elicited by 5-mV step depolarizations from a holding voltage of −90 mV or −100 mV, respectively.n=3–5, and error bars represent s.e.m. Descriptive values resulting from Boltzmann fits can be found in the Results section. (b) Recovery from fast inactivation of WT BgNav1 before (black), and after (red), addition of 1 μM rDc1a (red) determined by a double-pulse protocol to −30 mV with a varying time between pulses (0–50 ms). Values are reported in the Results section. Data representsn=4 experiments, and error bars represent the s.e.m. (c) On addition of 1 μM rDc1a to channels depolarized to −60 mV every 5 s (red open circles) or 50 s (green open circles; holding voltage was −100 mV), BgNav1-mediated sodium currents become rapidly visible. Channels completely recover after toxin washout. Inset shows current trace before (black), and after (red), addition of 1 μM rDc1a at −60 mV (5 s pulses). Noticeable is the persistent current that appears at this voltage, even in control experiments. Abscissa scale is 10 ms, ordinate scale is 0.3 μA. (d) Concentration dependence of rDc1a-induced current potentiation determined from shifts in the midpoint of channel activation (V1/2). Line represents a fit of the data with the Hill equation resulting in a half-maximal concentration (EC50) of 65±1 nM and a slope factor of 1.19±0.02;n=5 and error bars represent s.e.m. Figure 3: rDc1a promotes opening of BgNa v 1 channels. ( a ) Comparison of the gating properties of BgNa v 1 before (black), and after (red), addition of 1 μM rDc1a. Shown are the normalized deduced conductance ( G )–voltage (filled circles) ( G / G max ) and steady-state inactivation (open circles; I / I max ) relationships. Currents were elicited by 5-mV step depolarizations from a holding voltage of −90 mV or −100 mV, respectively. n =3–5, and error bars represent s.e.m. Descriptive values resulting from Boltzmann fits can be found in the Results section. ( b ) Recovery from fast inactivation of WT BgNa v 1 before (black), and after (red), addition of 1 μM rDc1a (red) determined by a double-pulse protocol to −30 mV with a varying time between pulses (0–50 ms). Values are reported in the Results section. Data represents n =4 experiments, and error bars represent the s.e.m. ( c ) On addition of 1 μM rDc1a to channels depolarized to −60 mV every 5 s (red open circles) or 50 s (green open circles; holding voltage was −100 mV), BgNa v 1-mediated sodium currents become rapidly visible. Channels completely recover after toxin washout. Inset shows current trace before (black), and after (red), addition of 1 μM rDc1a at −60 mV (5 s pulses). Noticeable is the persistent current that appears at this voltage, even in control experiments. Abscissa scale is 10 ms, ordinate scale is 0.3 μA. ( d ) Concentration dependence of rDc1a-induced current potentiation determined from shifts in the midpoint of channel activation (V 1/2 ). Line represents a fit of the data with the Hill equation resulting in a half-maximal concentration (EC 50 ) of 65±1 nM and a slope factor of 1.19±0.02; n =5 and error bars represent s.e.m. Full size image Interestingly, 1 μM rDc1a did not affect any of the tested vertebrate Na v channel isoforms or the hERG channel [34] , a member of the cardiac voltage-gated potassium (K v ) channel family and an Food and Drug Administration-mandated screening target for potential off-target drug effects ( Supplementary Fig. 2a ). These results are consistent with the report that Dc1a has no effect in mice when injected intraperitoneally or intracerebroventricularly at doses of 4.1 and 1.0 mg kg −1 , respectively [19] . rDc1a interacts with the domain II paddle motif in BgNa v 1 Subsequently, we were interested in identifying the receptor sites for rDc1a within insect Na v channels that result in such a profound shift in the voltage dependence of activation. Our experiments with BgNa v 1 suggest that rDc1a functions as an excitatory toxin to activate insect Na v channels at membrane voltages where they are normally closed. Hence, the toxin may interact with S3b–S4 paddle motifs within BgNa v 1 voltage sensors in a manner analogous to previously described β-scorpion toxins [3] , [35] , [36] . In order to test this hypothesis, we first needed to establish whether BgNa v 1 contains paddle motifs with similar functions as in K v channels [37] , [38] , [39] and in mammalian Na v channel isoforms where they have been identified (rNa v 1.2a, rNa v 1.4, rNa v 1.8, rNa v 1.9, and hNa v 1.9) [3] , [4] . To this end, we employed a previously reported approach in which specific S3b–S4 regions from each voltage-sensing domain of a Na v channel were transplanted into homotetrameric K v channels ( Fig. 4a ) [3] , [4] , [7] . After several attempts ( Fig. 4a ), we were able to generate functional chimeras between BgNa v 1 and K v 2.1 using known paddle motif boundaries [3] , [4] ( Fig. 4a,b ). All of the constructs contain the crucial basic residues that contribute to gating charge movement in K v channels [40] , [41] , suggesting that each of the four voltage-sensing domains in BgNa v 1 contain paddle motifs that are capable of sensing membrane voltage changes. 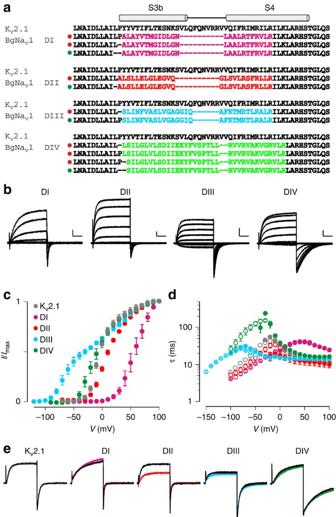Figure 4: Transfer of the voltage sensor paddle motifs from BgNav1 to Kv2.1. (a) Sequence alignment of the paddle region of Kv2.1 with the separate S3b–S4 regions of BgNav1 arranged per domain. In BgNav1, the paddle motifs are not identical and are therefore coloured differently: purple, domain I paddle (DI); red, domain II paddle (DII); blue, domain III paddle (DIII); green, domain IV paddle (DIV). In Kv2.1, the paddle motifs are identical and therefore have the same colour (black). Functional chimeras are indicated with a green dot in front of the sequence whereas non-functional chimeras are indicated with a red dot. (b,c) Transfer of the BgNav1 paddle motifs into Kv2.1. Families of potassium currents (b) and tail current voltage–activation relationships (c) for each chimeric construct (n=6; error bars represent s.e.m.). Holding voltage was −90 mV for DI, II, and IV, and −120 mV for DIII, and the tail voltage was −60 mV (−100 mV for DIII). Bars inbare 1 μA and 100 ms. (d) Kinetics of opening and closing for Kv2.1 channels containing paddle motifs from the four domains of BgNav1. Mean time constants (τ) from single-exponential fits to channel activation (filled circles) and deactivation (open circles) are plotted as a function of the voltage at which the current was recorded.n=6, and error bars represent s.e.m. (e) Potassium currents elicited by depolarizations near the foot (less than 1/3 of maximal activation) of the voltage–activation curve (c) for BgNav1/Kv2.1 chimeric constructs. Currents are shown before (black) and following (coloured) addition of 1 μM rDc1a. rDc1a clearly affects only the DII chimera. Figure 4: Transfer of the voltage sensor paddle motifs from BgNa v 1 to K v 2.1. ( a ) Sequence alignment of the paddle region of K v 2.1 with the separate S3b–S4 regions of BgNa v 1 arranged per domain. In BgNa v 1, the paddle motifs are not identical and are therefore coloured differently: purple, domain I paddle (DI); red, domain II paddle (DII); blue, domain III paddle (DIII); green, domain IV paddle (DIV). In K v 2.1, the paddle motifs are identical and therefore have the same colour (black). Functional chimeras are indicated with a green dot in front of the sequence whereas non-functional chimeras are indicated with a red dot. ( b , c ) Transfer of the BgNa v 1 paddle motifs into K v 2.1. Families of potassium currents ( b ) and tail current voltage–activation relationships ( c ) for each chimeric construct ( n =6; error bars represent s.e.m.). Holding voltage was −90 mV for DI, II, and IV, and −120 mV for DIII, and the tail voltage was −60 mV (−100 mV for DIII). Bars in b are 1 μA and 100 ms. ( d ) Kinetics of opening and closing for K v 2.1 channels containing paddle motifs from the four domains of BgNa v 1. Mean time constants ( τ ) from single-exponential fits to channel activation (filled circles) and deactivation (open circles) are plotted as a function of the voltage at which the current was recorded. n =6, and error bars represent s.e.m. ( e ) Potassium currents elicited by depolarizations near the foot (less than 1/3 of maximal activation) of the voltage–activation curve ( c ) for BgNa v 1/K v 2.1 chimeric constructs. Currents are shown before (black) and following (coloured) addition of 1 μM rDc1a. rDc1a clearly affects only the DII chimera. Full size image Examination of the conductance–voltage ( G – V ) relationships for the BgNa v 1/K v 2.1 chimeras reveals that each of the four voltage-sensor paddles has a distinct effect on the gating properties of K v 2.1. This was evidenced by marked differences in the midpoints of activation for the G – V relations for the domain I, II and IV constructs which are ⩾ 50 mV, 13±2 mV, and −9±2 mV, respectively ( Fig. 4c ). The G – V relationship for the domain III BgNa v 1/K v 2.1 construct is bimodal, suggesting that the functional coupling between the voltage-sensing domains and the pore has been considerably altered. Although the underlying mechanism is unclear, it is possible that pore opening in this particular chimera may occur when: (1) not all four voltage sensors are fully activated [42] ; or (2) each voltage sensor has transferred only a portion of its charge across the hydrophobic septum [43] , [44] , [45] . The latter scenario seems more likely since in the related Shaker K v channel, all four voltage sensor need to be in the active position before the pore opens [42] , [46] . Moreover, intermediate states have also been observed when measuring gating currents of the Shaker K v channel in which a mutation immobilized voltage-sensor movement between the resting and activated states, thereby shifting the voltage activation of the ionic currents [47] . Finally, it is worth mentioning that the domain III BgNa v 1/K v 2.1 construct may display multiple open states according to a model that has been described for N-type Ca v channels [48] . Remarkably, domain IV paddle motifs from rNa v 1.2a and rNa v 1.4 slow activation kinetics when transplanted into K v channels. These observations support the notion that the domain IV paddle motif contributes substantially to the overall rate of voltage-sensor activation [3] , [4] . To explore whether the domain IV paddle motif serves a similar role in BgNa v 1, we measured the kinetics of activation and deactivation of the four BgNa v 1 paddle constructs in response to membrane depolarization and repolarization, respectively. Similar to previously studied chimeric channels, the activation and deactivation kinetics observed for the domain IV construct of BgNa v 1/K v 2.1 are slower over a wide voltage range when compared with the other domains ( Fig. 4d ), suggesting that this particular domain may indeed contribute to fast inactivation in insect Na v channels [49] , [50] , [51] . We obtained additional evidence for the functional role of the domain IV paddle motif in BgNa v 1 gating from experiments with BomIV, a classic insect-selective α-scorpion toxin from the venom of Buthus occitanus mardochei that inhibits fast inactivation in American cockroach neurons [52] . To determine whether BomIV influences BgNa v 1 in a similar fashion, we applied 10 nM to channel-expressing Xenopus oocytes and observed that the toxin indeed slows down fast inactivation ( Supplementary Fig. 2b ). Subsequent testing on the BgNa v 1/K v 2.1 chimeras revealed that BomIV does not affect WT K v 2.1 or the domain I, II, and III constructs. However, a dramatic toxin-induced inhibition of the domain IV chimera corroborates the importance of this particular voltage-sensing domain in toxin binding and BgNa v 1 fast inactivation ( Supplementary Fig. 2b ). We next investigated whether rDc1a modulates the activity of any of the four BgNa v 1/K v 2.1 paddle chimeras and found that 1 μM rDc1a exclusively interacts with the domain II construct whereas domains I, III, IV, and WT K v 2.1 are unaffected ( Fig. 4e , Supplementary Fig. 2c ). This result suggests that rDc1a specifically targets the domain II voltage sensor within BgNa v 1 to influence channel opening. rDc1a distinguishes between cockroach Na v 1 channels Since the domain II paddle motif in BgNa v 1 (ref. 21 ) is identical to that in PaNa v 1 (ref. 22 ), we expected a similar effect of rDc1a in whole-cell patch-clamp recordings from American cockroach dorsal unpaired median (DUM) neurons. Surprisingly, 1μM rDc1a had little effect on sodium current amplitude or kinetics in DUM neurons as reflected in the threshold, or V 1/2 , of Na v channel activation or the V 1/2 of steady-state inactivation measurements ( Supplementary Fig. 3 ). Furthermore, there were no significant use-dependent effects on sodium current amplitude or kinetics. Due to the unexpectedly weak effects of 1μM rDc1a on voltage-dependent activation of P. americana DUM neurons compared with BgNa v 1 channels from B. germanica , acute toxicity assays were expanded to include both cockroach species ( Fig. 5a,b ). Remarkably, these bioassays revealed lethal toxicity of rDc1a in B. germanica compared with only mild, reversible effects in P. americana . At doses up to 5 nmol g −1 , rDc1a generated only minor spastic contractions of the abdomen, some shaking and evidence of reduced motor activity in P. americana . Even though these effects were completely reversible, a very small percentage of cockroaches did develop paralysis after 24 h (7±7% knockdown, n =3). One explanation for these observations may be toxin binding to a subset of Na v channel splice variants [53] or the presence of endogenous pharmacologically active auxiliary subunits [54] . Conversely, B. germanica underwent dose-dependent flaccid or contractile paralysis, and lethality was observed after 8 h at all doses tested ( Fig. 5a ). The KD 50 and LD 50 values at 24 h post injection were 3.0±1.2 nmol g −1 and 4.2±3.4 nmol g −1 ( n =3), respectively. These observations suggest that residues in regions outside of the domain II paddle motif may underlie the remarkably different sensitivity of BgNa v 1 and PaNa v 1 to rDc1a. 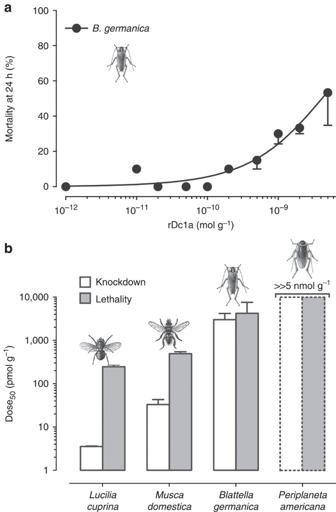Figure 5: Acute toxicity of rDc1a in two cockroach families. (a) Dose–response curve for lethal effects of rDc1a determined 24 h after injection into German cockroaches (B. germanica; family Blattellidae, closed circles). Data were fitted according to Equation 5 in Methods and represent mean±s.e.m. of three independent experiments. (b) Comparison of the KD50(open columns) and LD50(grey columns) doses at 24 h following injection of rDc1a inL. cuprina,M. domesticaandB. germanica. Note: doses up to 5 nmol g−1failed to produce any signs of knockdown or lethality up to 72 h post injection in American cockroaches (Periplaneta americana; family Blattidae). Data represent mean±s.e.m. of three independent experiments. Figure 5: Acute toxicity of rDc1a in two cockroach families. ( a ) Dose–response curve for lethal effects of rDc1a determined 24 h after injection into German cockroaches ( B. germanica ; family Blattellidae, closed circles). Data were fitted according to Equation 5 in Methods and represent mean±s.e.m. of three independent experiments. ( b ) Comparison of the KD 50 (open columns) and LD 50 (grey columns) doses at 24 h following injection of rDc1a in L. cuprina , M. domestica and B. germanica . Note: doses up to 5 nmol g −1 failed to produce any signs of knockdown or lethality up to 72 h post injection in American cockroaches ( Periplaneta americana ; family Blattidae). Data represent mean±s.e.m. of three independent experiments. Full size image The S1–S2 loop modulates Na v channel sensitivity to rDc1a Sequence alignment of BgNa v 1 with PaNa v 1 reveals a highly conserved S1–S4 voltage sensor in domain II with only three amino acid substitutions ( Fig. 6a ; Supplementary Fig. 4 ). Of those, two residues in the S1–S2 loop are potentially accessible for a peptide toxin applied from the extracellular environment (His805 and Asp812 in BgNa v 1 which correspond to a Tyr and Glu in PaNa v 1, respectively). On mutating these residues in BgNa v 1 to their PaNa v 1 counterparts, the resulting BgNa v 1 YE construct functionally expressed in Xenopus oocytes with a voltage-dependent activation V 1/2 of −41.5±0.3 mV and a steady-state inactivation V 1/2 of −56.4±0.2 mV ( Fig. 6b ). Unfortunately, a functional PaNa v 1 clone was unavailable to undertake gain-of-function experiments. Strikingly, 100 nM rDc1a was no longer sufficient to open BgNa v 1 YE whereas this concentration generated large inward sodium currents when applied to WT channels ( Fig. 6c , inset). When surveying higher concentrations of rDc1a, it becomes clear that concentrations of more than 1 μM are required to achieve a potentiation with BgNa v 1 YE that is comparable to the WT channel (EC 50 ~65 nM; Fig. 6c ). Although we cannot exclude the possibility that rDc1a interacts with other PaNa v 1 domains at such concentrations, administering high doses of the toxin is indeed mildly toxic to P. americana ( Fig. 5a,b ). Thus, our mutagenesis experiments have uncovered a novel region within insect Na v channels that helps determine their sensitivity to spider toxins. This locus contributes to the drastically reduced sensitivity of the American cockroach to rDc1a from the venom of the desert bush spider whereas its German counterpart is highly susceptible. 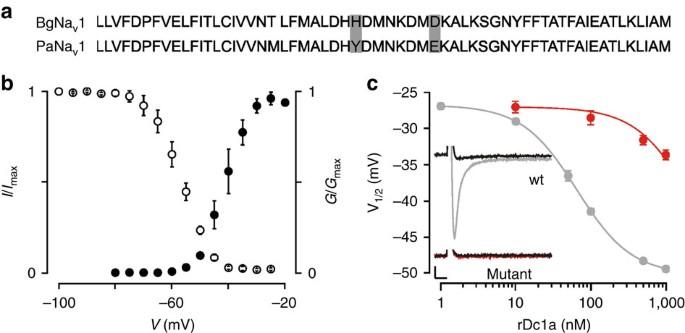Figure 6: Residues outside of the DII paddle motif contribute to rDc1a binding. (a) Sequence alignment of the DII S1–S2 regions of BgNav1 and PaNav1 (SeeSupplementary Fig. 4for more details). In the extracellular loop connecting S1 to S2, all residues are identical except the H805Y and D812E substitutions (grey background). The T797M substitution within S1 is unlikely to be toxin-accessible. (b) Gating properties of the mutant BgNav1YEchannel. Shown are the normalized deduced conductance (G)–voltage (filled circles) (G/Gmax) and steady-state inactivation (open circles;I/Imax) relationships. Descriptive values can be found in the Results section. Currents were elicited by 5 mV step depolarizations from a holding voltage of −90 mV or −100 mV, respectively.n=3–5, and error bars represent s.e.m. (c) Affinity measure for rDc1a interaction with BgNav1YE(red) compared with WT BgNav1 (grey). Concentration dependence for toxin-induced current potentiation (as determined by shifts in V1/2) is shown. It is clear that alterations in channel opening on rDc1a exposure are less pronounced with the BgNav1YEmutant when compared with WT BgNav1.n=5 and error bars represent s.e.m. Inset shows premature channel opening after addition of 100 nM rDc1a to WT BgNav1 (grey) whereas BgNav1YEis not yet affected (red). Current traces were evoked by a 50-ms depolarization to −55 mV from a holding potential of −90 mV. Figure 6: Residues outside of the DII paddle motif contribute to rDc1a binding. ( a ) Sequence alignment of the DII S1–S2 regions of BgNa v 1 and PaNa v 1 (See Supplementary Fig. 4 for more details). In the extracellular loop connecting S1 to S2, all residues are identical except the H805Y and D812E substitutions (grey background). The T797M substitution within S1 is unlikely to be toxin-accessible. ( b ) Gating properties of the mutant BgNa v 1 YE channel. Shown are the normalized deduced conductance ( G )–voltage (filled circles) ( G / G max ) and steady-state inactivation (open circles; I / I max ) relationships. Descriptive values can be found in the Results section. Currents were elicited by 5 mV step depolarizations from a holding voltage of −90 mV or −100 mV, respectively. n =3–5, and error bars represent s.e.m. ( c ) Affinity measure for rDc1a interaction with BgNa v 1 YE (red) compared with WT BgNa v 1 (grey). Concentration dependence for toxin-induced current potentiation (as determined by shifts in V 1/2 ) is shown. It is clear that alterations in channel opening on rDc1a exposure are less pronounced with the BgNa v 1 YE mutant when compared with WT BgNa v 1. n =5 and error bars represent s.e.m. Inset shows premature channel opening after addition of 100 nM rDc1a to WT BgNa v 1 (grey) whereas BgNa v 1 YE is not yet affected (red). Current traces were evoked by a 50-ms depolarization to −55 mV from a holding potential of −90 mV. Full size image The initial goal of this study was to explore the mechanism underlying the efficacy of Dc1a, a potent insecticidal peptide toxin produced by desert bush spiders. To this end, we first produced recombinant rDc1a and determined its solution structure using heteronuclear NMR ( Figs 1 and 2 ). Next, we tested rDc1a on the heterologously expressed German cockroach channel BgNa v 1 and discovered that the toxin dramatically promotes channel opening ( Fig. 3 ). By taking advantage of the portable nature of S3b–S4 paddle motifs within voltage-sensing domains [3] , [4] , [7] , [38] , we demonstrated that such motifs also exist in each of the four voltage-sensing domains of BgNa v 1, and that rDc1a selectively interacts with the paddle motif in domain II, a feature that it shares with an extensive list of animal toxins that target this particular paddle motif [3] , [4] , [12] , [55] , [56] , albeit with a high degree of insect selectivity ( Fig. 4 ). Remarkably, our insect assays revealed that German cockroaches are highly susceptible to rDc1a whereas the closely related American cockroach is virtually insensitive despite the fact that the domain II paddle motif in BgNa v 1 is identical to that in PaNa v 1 ( Fig. 5 ; Supplementary Fig. 4 ). To elucidate the machinery responsible for this discrepancy, we mutated two residues in the S1–S2 loop that differ between BgNa v 1 and PaNa v 1 (His805 and Asp812) and found that the susceptibility of the resulting BgNa v 1 YE construct to rDc1a is dramatically reduced ( Fig. 6 ). Interestingly, mammalian Na v channel isoforms possess a Tyr and Ser at the corresponding positions, which presumably contributes to their insensitivity to rDc1a; however, their domain II paddle motif differs as well ( Supplementary Fig. 4 ). It is interesting to consider potential mechanisms that may underlie the insect-family specificity of rDc1a. For example, the β3–β4 hairpin ( Fig. 2b ) often houses the pharmacophore in spider ICK toxins that target voltage-gated ion channels [57] , but the unusual architecture of rDc1a ( Fig. 2c ) and its unique ability to dramatically promote opening of insect Na v channels ( Fig. 3 ) suggests that it might interact with the voltage sensors of these channels in a unique manner. As such, the domain II S1–S2 loop may play a role in positioning the toxin into a water-filled cavity adjacent to the S3–S4 paddle motif [58] , thereby placing particular toxin residues in strategic positions to stabilize the domain II voltage sensor in an activated position. This hypothesis is strengthened by the observation that the substitution of two residues in the domain II S1–S2 loop within mammalian Na v 1.2 channels decreases sensitivity to the functionally related β-scorpion toxin CssIV by a factor of four [59] . Another possible mechanism is that rDc1a binding to the domain II S1–S2 loop in BgNa v 1 allosterically influences channel opening. Such a hypothesis was postulated when a domain III S1 splice variant of BgNa v 1 revealed an increased susceptibility to the insect-selective β-scorpion toxin Lqh-dprIT 3 (ref. 60 ). However, one caveat is that a depolarizing prepulse is needed to potentiate the maximal effect of CssIV and Lqh-dprIT 3 (refs 49 , 50 ). Similar to the structurally unrelated spider toxin Magi5 which activates rat Na v 1.2 channels by binding to the domain II voltage sensor [61] , rDc1a does not require such a prepulse. In summary, the current study provides a molecular explanation for the remarkable insect selectivity of Dc1a, the most potent insecticidal toxin identified in the venom of the desert bush spider. Moreover, we have uncovered a novel toxin receptor site within insect Na v channels that provides a new framework for the design of molecules capable of targeting specific insect families. This knowledge may be used in the future to develop insecticides that target specific insect pests without affecting beneficial insects or endangering human health. Chemicals All chemicals were purchased from Sigma-Aldrich Australia (Castle Hill, NSW, Australia), Sigma-Aldrich USA (St Louis, MO, USA), or Merck Chemicals (Kilsyth, Victoria, Australia) with the exception of IPTG and streptomycin (Life Technologies, Victoria, Australia), tetrodotoxin (Alomone Labs, Israel), and high-performance liquid chromatography (HPLC)-grade acetonitrile (RCI Labscan, Bangkok, Thailand). 13 C 6 -glucose and 15 NH 4 Cl were from Sigma-Aldrich Australia. Recombinant His 6 -TEV protease (EC 3.4.22.44) was produced in-house using a published protocol [62] . Production of recombinant rDc1a A synthetic gene encoding Dc1a, with codons optimized for expression in Escherichia coli , was produced and cloned into a variant of the pLIC-MBP expression vector by GeneArt (Invitrogen, Regensburg, Germany). This vector (pLIC-NSB3) encodes a MalE signal sequence for periplasmic export, a His 6 tag for affinity purification, a maltose-binding protein (MBP) fusion tag to aid solubility, and a tobacco etch virus (TEV) protease recognition site directly preceding the codon-optimized Dc1a gene [23] . The plasmid encoding Dc1a was transformed into E. coli strain BL21(λDE3) for recombinant toxin production. Protein expression and purification were performed as described previously [30] with minor modifications. In summary, cultures were grown in Luria-Bertani broth at 37 °C with shaking. Toxin gene expression was induced with 500 μM IPTG at an OD 600 of 1.0–1.1, then cells were grown at 20 °C for a further 12 h before collecting by centrifugation for 15 min at 10,500 g . For production of uniformly 13 C/ 15 N-labelled rDc1a, cultures were grown in minimal medium supplemented with 13 C 6 -glucose and 15 NH 4 Cl as the sole carbon and nitrogen sources, respectively. The His 6 -MBP-toxin fusion protein was extracted from the bacterial periplasm by cell disruption at 27 kPa (TS Series Cell Disrupter, Constant Systems Ltd, Northants, UK), and then captured by passing the extract (buffered in 40 mM Tris, 450 mM NaCl, pH 8.0) over Ni-NTA Superflow resin (Qiagen, Chadstone, Australia). Proteins bound non-specifically were removed by washing with 10 mM imidazole then the fusion protein was eluted with 600 mM imidazole. The eluted fusion protein was concentrated to 10 ml and the buffer was exchanged to remove imidazole. Reduced and oxidized glutathione were then added to a final concentration of 0.6 mM and 0.4 mM, respectively, to maintain TEV protease activity and promote folding of the protein. Approximately, 100 μg of His 6 -tagged TEV protease was added per mg of rDc1a, then the cleavage reaction was allowed to proceed at room temperature for 12 h. The cleaved His 6 -MBP and His 6 -TEV were precipitated by addition of 1% trifluoroacetic acid (TFA), then the sample was centrifuged at 16,000 g . The supernatant was filtered using a 0.45-μm syringe filter (Millipore, MA, USA) and subjected to further purification using RP-HPLC. RP-HPLC was performed on a Vydac C18 column (250 × 4.6 mm, particle size 5 μm) using a flow rate of 1 ml min −1 and a gradient of 20–45% Solvent B (0.043% TFA in 90% acetonitrile) in Solvent A (0.05% TFA in water) over 30 min. rDc1a contains a non-native N-terminal serine residue (a vestige of the TEV protease cleavage site), making it one residue longer than native Dc1a. Mass spectrometry Toxin masses were confirmed by MALDI-TOF mass spectrometry using a Model 4700 Proteomics Bioanalyser (Applied Biosystems, CA, USA). RP-HPLC fractions were mixed (1:1 v-v) with α-cyano-4 hydroxycinnamic acid matrix (5 mg ml −1 in 50/50 acetonitrile/H 2 O) and MALDI-TOF spectra were acquired in positive reflector mode. All reported masses are for monoisotopic [M+H] + ions. Structure determination Several buffer conditions were screened to optimize quality of NMR data recorded for rDc1a, including 20 mM phosphate buffer, pH 6.0; 20 mM MES buffer, pH 6.0 and 20 mM acetate buffer pH 5.0. Initial buffer screening revealed the acetate buffer, pH 5.0 was optimal for acquisition of NMR data. Recombinant 15 N/ 13 C-labelled rDc1a was dissolved in 20 mM acetate buffer, pH 5.0 to a final concentration of 350 μM. 5% 2 H 2 O was added, then the sample was filtered using a low-protein-binding Ultrafree-MC centrifugal filter (0.22 μm pore size; Millipore, MA, USA) and 300 μl was added to a susceptibility matched 5 mm outer-diameter microtube (Shigemi Inc., Japan). NMR data were acquired at 25 °C using a 900 MHz NMR spectrometer (Bruker BioSpin, Germany) equipped with a cryogenically cooled probe. 3D and 4D data used for resonance assignments were acquired using non-uniform sampling. Sampling schedules that approximated the signal decay in each indirect dimension were generated using sched3D [26] . Non-uniform sampling data were processed using the Rowland NMR toolkit ( www.rowland.org/rnmrtk/toolkit.html ) and maximum entropy parameters were automatically selected as previously described [63] . 13 C- and 15 N-edited HSQC-NOESY (mixing time of 200 ms) experiments were acquired using uniform sampling. All experiments were acquired in H 2 O containing 5% 2 H 2 O. Dihedral angles (φ, ψ) were derived from TALOS+chemical shift analysis [64] and the restraint range for structure calculations was set to twice the estimated s.d. The Gly9–Pro10 and Arg36–Pro37 peptide bond was determined to be in the trans conformation on the basis of characteristic NOEs and the C α and C β chemical shifts of Pro residues. NOESY spectra were manually peak picked and integrated, then peak lists were automatically assigned, distance restraints extracted and an ensemble of structures calculated using the torsion angle dynamics package CYANA 3.0 (ref. 25 ). The tolerances used for CYANA 3.0 were 0.025 p.p.m. in the direct 1 H dimension, 0.03 p.p.m. in the indirect 1 H dimension and 0.3 p.p.m. for the heteronucleus ( 13 C/ 15 N). During the automated NOESY assignment/structure calculation process, CYANA assigned 92% of all NOESY crosspeaks (2,271 out of 2,469). Insecticidal assays rDc1a was dissolved in insect saline and injected into the ventro-lateral thoracic region of adult sheep blowflies ( Lucilia cuprina ;), adult houseflies ( M. domestica ), adult American cockroaches ( Periplaneta americana ) and adult German cockroaches ( Blattella germanica ) [65] . Injections were made using a 1.0 ml Terumo Insulin syringe (B-D Ultra-Fine, Terumo Medical Corporation, Maryland, USA) with a fixed 29 G needle fitted to an Arnold hand micro-applicator (Burkard Manufacturing Co. Ltd., England). A maximum volume of 2 μl was injected per L. cuprina, M. domestica and B. germanica and 5 μl for the larger P. americana . Thereafter, flies were individually housed in 2-ml tubes and provided with 10% sucrose while cockroaches were housed in closed Petri dishes and provided with dry food and water. The paralytic activity was then determined over a 24-h period. For each acute toxicity assay up to fourteen doses of rDc1a ( n =10 insects per dose) and the appropriate control (insect saline; n =10 insects) were used. The assay was repeated three times. Median knockdown (KD 50 ) and median lethal (LD 50 ) doses were calculated as described previously [66] and averaged to produce KD 50 and LD 50 values. Electrophysiological measurements on DUM neurons DUM neurons were isolated from unsexed adult American cockroaches ( P. americana ) as described previously [30] . Briefly, terminal abdominal ganglia were removed and placed in normal insect saline (NIS) containing (in mM): NaCl 180, KCl 3.1, N -hydroxyethylpiperazine- N -ethanesulfonic acid (HEPES) 10 and D-glucose 20. Ganglia were then incubated in 1 mg ml −1 collagenase (type IA) for 40 min at 29 °C. Following enzymatic treatment, ganglia were washed three times in NIS and triturated through a fire-polished Pasteur pipette. The resultant cell suspension was then distributed onto 12-mm diameter glass coverslips pre-coated with 2 mg ml −1 concanavalin A (type IV). DUM neurons were maintained in NIS supplemented with 5 mM CaCl 2 , 4 mM MgCl 2 , 5% foetal bovine serum and 1% penicillin and streptomycin (Life Technologies, Victoria, Australia), and maintained at 29 °C, 100% humidity. Ionic currents were recorded in voltage-clamp mode using the whole-cell patch-clamp technique employing version 10.2 of the pCLAMP data acquisition system (Molecular Devices, Sunnyvale, CA). Data were filtered at 5–10 kHz with a low-pass Bessel filter with leakage and capacitive currents subtracted using P-P /4 procedures. Digital sampling rates were set between 15 and 25 kHz depending on the length of the protocol. Single-use 0.8–2.5 MΩ electrodes were pulled from borosilicate glass and fire-polished prior to current recordings. Liquid junction potentials were calculated using JPCALC, and all data were compensated for these values. Cells were bathed in external solution through a continuous pressurized perfusion system at 1 ml min −1 , while toxin solutions were introduced via direct pressurized application via a perfusion needle at ~ 50 μl min −1 (Automate Scientific, San Francisco, CA). Control data were not acquired until at least 20 min after whole-cell configuration was achieved to eliminate the influence of initially fast time-dependent shifts in steady-state inactivation resulting in Na V channel current ( I Na ) rundown. All experiments were performed at ambient temperature (20–23 °C). To record I Na , the external bath solution contained (in mM): NaCl 80, CsCl 5, CaCl 2 1.8, tetraethylammonium chloride 50, 4-aminopyridine 5, HEPES 10, NiCl 2 0.1, and CdCl 2 1, adjusted to pH 7.4 with 1 M NaOH. The pipette solution contained (in mM): NaCl 34, CsF 135, MgCl 2 1, HEPES 10, ethylene glycol-bis(2-aminoethylether)- N , N , N ′, N ′-tetraacetic acid 5, and ATP-Na 2 3, adjusted to pH 7.4 with 1 M CsOH. To eliminate any influence of differences in osmotic pressure, all internal and external solutions were adjusted with sucrose to 400±5 mOsmol l −1 . Experiments were rejected if there were large leak currents or currents showed signs of poor space clamping. Off-line data analysis was performed using Axograph X version 1.3 or Clampfit 10 (Molecular Devices, USA). Voltage–activation relationships were obtained by measuring steady-state currents elicited by stepwise depolarizations of 5–10 mV from a holding potential of –90 mV and calculating peak conductance ( G Na ) using the following equation: G = I Na /( V m – E rev ) where G is peak conductance, I Na is peak inward sodium current, V m is the test potential and E rev is the reversal potential. Reversal potentials were individually estimated for each data set [67] by fitting the I Na - V data with the following equation: I Na =[1+exp(–0.03937 × z × ( V m –V 1/2 ))] −1 × g × ( V m – V rev ) where z is the apparent gating charge, g is a factor related to the number of channels contributing to the macroscopic whole-cell I Na , V m is equal to the voltage potential of the pulse, and V 1/2 is the voltage at half-maximal activation. The normalized conductance was fitted to a two-state Boltzmann function of the form: G / G max =1/(1+exp((–0.3937 × z × ( V m – V 1/2 ))) where G , z, V m and V 1/2 have the same meaning. The voltage dependence of steady-state Na v channel inactivation ( h ∞ /V ) data were normalized to the maximum peak current in the control or maximum peak current and fitted using the following Boltzmann equation: h ∞ =A/(1+exp(( V m – V 1/2 )/ k )) where A is the fraction of control maximal peak I Na (value of 1.0 under control conditions), V 1/2 is the midpoint of steady-state inactivation, k is the slope factor and V m is the prepulse voltage. The rate of recovery from fast inactivation data were fitted to the following single-exponential function: I / I max =1−exp(– τ / t ) where τ is the time constant of current recovery. Dose–response curves to determine LD 50 and KD 50 values were fitted using the following form of the logistic equation: y =1/(1+[ x ]/Dose 50 ) n H where x is the toxin dose, n H the Hill coefficient (slope parameter) and Dose 50 is the median inhibitory dose causing lethality (LD 50 ) or knockdown (KD 50 ). Non-linear curve-fitting of data were performed using GraphPad Prism version 6.00c for Macintosh (GraphPad Software, San Diego) or Origin 8 (OriginLab, MA, USA). Comparisons of two sample means were made using a paired Student’s t -test and differences were considered to be significant if P <0.05. All data are presented as mean±s.e.m. of n independent experiments. Electrophysiological measurements on oocytes Chimeras and channel mutants were generated using sequential PCRs with K v 2.1Δ7 (ref. 68 ) and BgNa v 1 (ref. 21 ) as templates. The Kv2.1Δ7 construct contains seven point mutations in the outer vestibule, rendering the channel sensitive to agitoxin-2. The DNA sequence of all constructs and mutants was confirmed by automated DNA sequencing and cRNA was synthesized using T7 polymerase (mMessage mMachine kit, Life Technologies, USA) after linearizing the DNA with appropriate restriction enzymes. Channel constructs including hNa v 1.1–hNa v 1.7 and hERG were expressed in Xenopus oocytes by themselves or, in the case of BgNa v 1, together with the TipE subunit [69] (1:5 molar ratio), and studied following 1–2 days incubation after cRNA injection (incubated at 17 °C in 96 mM NaCl, 2 mM KCl, 5 mM HEPES, 1 mM MgCl 2 and 1.8 mM CaCl 2 , 50 μg ml −1 gentamycin, pH 7.6 with NaOH) using two-electrode voltage-clamp recording techniques (OC-725C, Warner Instruments, USA) with a 150-μl recording chamber. Data were filtered at 4 kHz and digitized at 20 kHz using pClamp software (Molecular Devices, USA). Microelectrode resistances were 0.5–1 MΩ when filled with 3 M KCl. For most K v channel experiments, the external recording solution contained (in mM): 50 KCl, 50 NaCl, 5 HEPES, 1 MgCl 2 , 0.3 CaCl 2 , pH 7.6 with NaOH. For Na v channel experiments, the external recording solution contained (in mM): 96 NaCl, 2 KCl, 5 HEPES, 1 MgCl 2 and 1.8 CaCl 2 , pH 7.6 with NaOH. All experiments were performed at room temperature (~22 °C). Leak and background conductances, identified by blocking the channel with agitoxin-2 (Alomone labs) or tetrodotoxin, were subtracted for most of the K v or BgNa v 1 currents shown. Voltage–activation relationships were obtained by measuring tail currents for K v channels or steady-state currents and calculating conductance for Na v channels. Protocols for other measurements are described in the figure legends. After addition of the toxin to the recording chamber, the equilibration between the toxin and the channel was monitored using weak depolarizations elicited at 5-s intervals. For all channels, we recorded voltage–activation relationships in the absence and presence of toxin. Off-line data analysis was performed using Clampfit 10 (Molecular Devices, USA), Origin 8.0 (Originlab) and Microsoft Solver (Microsoft Excel). How to cite this article: Bende, N. S. et al . A distinct sodium channel voltage-sensor locus determines insect selectivity of the spider toxin Dc1a. Nat. Commun. 5:4350 doi: 10.1038/ncomms5350 (2014). Accession codes : Complete chemical shift assignments for rDc1a have been deposited in BioMagResBank under accession code 19666 .